Autophagic degradation of the inhibitory p53 isoform Δ133p53α as a regulatory mechanism for p53-mediated senescence Δ133p53α, a p53 isoform that can inhibit full-length p53, is downregulated at replicative senescence in a manner independent of mRNA regulation and proteasome-mediated degradation. Here we demonstrate that, unlike full-length p53, Δ133p53α is degraded by autophagy during replicative senescence. Pharmacological inhibition of autophagy restores Δ133p53α expression levels in replicatively senescent fibroblasts, without affecting full-length p53. The siRNA-mediated knockdown of pro-autophagic proteins (ATG5, ATG7 and Beclin-1) also restores Δ133p53α expression. The chaperone-associated E3 ubiquitin ligase STUB1, which is known to regulate autophagy, interacts with Δ133p53α and is downregulated at replicative senescence. The siRNA knockdown of STUB1 in proliferating, early-passage fibroblasts induces the autophagic degradation of Δ133p53α and thereby induces senescence. Upon replicative senescence or STUB1 knockdown, Δ133p53α is recruited to autophagosomes, consistent with its autophagic degradation. This study reveals that STUB1 is an endogenous regulator of Δ133p53α degradation and senescence, and identifies a p53 isoform-specific protein turnover mechanism that orchestrates p53-mediated senescence. Autophagy is an evolutionarily conserved system for degrading long-lived proteins, aggregated proteins, damaged organelles and certain pathogens [1] . While a low level of basal autophagy is responsible for homeostatic control of protein and organelle quality under non-stress conditions, nutrient starvation or cellular stress dramatically induces autophagy for non-selective bulk degradation, which recycles cellular components for essential metabolism and stress response [1] , [2] . Recent evidence suggests that, in addition to this non-selective bulk autophagy, a process termed ‘selective autophagy’ targets specific sets of ubiquitinated substrates [3] , [4] , functioning as a ubiquitin-dependent degradation mechanism alternative to proteasome-mediated degradation. The autophagy machinery comprises various pro-autophagic proteins functioning in phagophore formation, autophagosome formation and autophagosome–lysosome fusion. These include a set of autophagy-related (ATG) proteins such as ATG5, ATG12 and ATG7 (the former two forming conjugates through the activity of the latter) [5] ; Beclin-1 (also called ATG6), a component of the Vps34 complex [6] ; and a lipid-conjugated form of microtubule-associated protein 1 light chain 3 (LC3-II), an autophagosome protein whose turnover serves as an index of autophagy flux [7] , [8] . p62/SQSTM1 enters into autophagosomes through binding to LC3-II and is degraded as an autophagy substrate; it also functions as a ubiquitin-binding receptor for other ubiquitinated substrates to be incorporated into autophagosomes and degraded by selective autophagy [3] , [4] , [9] . Autophagy is suggested to contribute to the regulation of aging in various model organisms from yeast to mammals: overall inhibition of basal autophagic activity (for example, due to defective Beclin-1 or ATG proteins) is associated with accelerated aging phenotypes and shortened lifespan [10] , [11] , [12] . Conversely, enhanced basal autophagy (for example, due to transgenic expression of ATG proteins or administration of rapamycin) can delay aging and extend lifespan [11] , [13] , [14] . Autophagy is also implicated in cancer and a wide variety of other disorders [15] . Autophagy seems to play dual roles in carcinogenesis: basal or stress-induced autophagy in normal cells serves as a barrier to suppress tumour initiation by limiting reactive oxygen species production, inflammation, tissue damage and genome instability; once cancer is established, however, high levels of basal autophagy contribute to cancer cell survival under hypoxia and metabolic stress [2] , [16] , [17] . Despite these accumulating findings, the role of selective autophagy during aging and carcinogenesis is largely unknown, and specific autophagy substrates involved in these processes remain to be identified. Another well-known cellular phenotype contributing to aging and carcinogenesis is cellular senescence, a state of sustained proliferation arrest [18] , [19] , and functional interplays between cellular senescence and autophagy have been reported in various cell types including starved plants [20] and human cells [21] . Cellular senescence is triggered by telomere dysfunction resulting from extensive cell divisions (replicative senescence) [22] , illegitimate activation of oncogenes (oncogene-induced senescence) [23] , [24] or other types of cellular stresses [25] , [26] . The tumour suppressor protein p53 and its interacting pathways play key roles in signalling these cellular stresses [19] , [27] . A growing body of evidence suggests that functionally distinct p53 protein isoforms, which arise because of alternative mRNA splicing or alternative promoter usage, modulate the biological processes regulated by full-length p53 protein [28] , [29] . We and others [28] , [30] previously reported that Δ133p53α, a p53 isoform that lacks the N-terminal region responsible for transactivation and interaction with MDM2 (ref. 31 ), dominant-negatively inhibits the activity of full-length p53, while this isoform is also suggested to function in a promoter-specific manner and independently of full-length p53 (ref. 32 ). Endogenous Δ133p53α protein was found to be downregulated during replicative senescence, but not upon oncogene-induced senescence, in human fibroblasts [30] . Knockdown or overexpression of Δ133p53α induced or delayed replicative senescence through the regulation of p53 target genes, suggesting a physiological role of this p53 isoform in replicative senescence [30] . The downregulation of Δ133p53α at replicative senescence was not because of a change in mRNA levels [30] . Unlike full-length p53 protein that is subject to proteasomal degradation, Δ133p53α was not stabilized by treatment with the proteasome inhibitor MG-132 (ref. 30 ). These findings prompted us to investigate whether the protein turnover of Δ133p53α is controlled by autophagy as an alternative mechanism. This study shows that an isoform-specific degradation mechanism constitutes a p53-regulated biological process and suggests that Δ133p53α represents a functional and regulatory link between cellular senescence and autophagy, two cellular phenotypes involved in aging and cancer. Pharmacological inhibition of autophagy restores Δ133p53α To examine the kinetics of protein turnover of endogenous Δ133p53α in normal human cells, protein synthesis was blocked by cycloheximide treatment in MRC-5 fibroblasts and the amounts of Δ133p53α protein were monitored ( Fig. 1a ). In contrast to full-length p53, which decreased over time, the amounts of Δ133p53α were dramatically increased at 3 and 6 h, making it impossible to determine the half-life of Δ133p53α in this experiment. This result instead suggested that the degradation of endogenous Δ133p53α in normal human fibroblasts required a protein (or proteins) with a rapid turnover rate, which is reminiscent of autophagic protein degradation [33] , [34] . The phosphoinositide 3-kinase inhibitors wortmannin and LY294002, which inhibit autophagy [35] , but not an inactive analogue LY303511 (ref. 36 ), increased the amounts of Δ133p53α protein in MRC-5 fibroblasts ( Fig. 1b ), providing further indication for autophagic degradation of Δ133p53α. 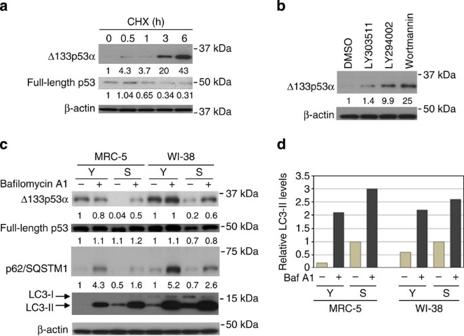Figure 1: Pharmacological inhibition of autophagy restores Δ133p53α expression. (a) Δ133p53α expression is induced by cycloheximide (CHX). MRC-5 fibroblasts (at population doubling levels (PDLs) 51) were treated with CHX (25 μg ml−1) for indicated time periods and examined in immunoblot for Δ133p53α and full-length p53. β-actin was a loading control for normalization. The relative expression levels of Δ133p53α and full-length p53 are shown below the images. (b) Δ133p53α expression is induced by phosphoinositide 3-kinase inhibitors. MRC-5 fibroblasts (PDLs 51) were treated for 4 h with LY303511 (10 μM), LY294002 (10 μM), Wortmannin (50 nM) or dimethylsulphoxide alone (as control) and examined in immunoblot for Δ133p53α and β-actin expression. (c) Diminished Δ133p53α at replicative senescence is restored by treatment with bafilomycin A1. The immunoblot analyses were performed in early-passage (Y) and replicatively senescent (S) human fibroblast strains MRC-5 and WI-38. The examined PDLs were 30 (Y) and 60 (S) for MRC-5; and 30 (Y) and 54 (S) for WI-38. Bafilomycin A 1 treatment was at 100 nM for 4 h. The relative expression levels of Δ133p53α, full-length p53 and p62/SQSTM1 (normalized with β-actin) are shown. Anti-LC3B antibody detected LC3-I and LC3-II, which was used in quantitative analysis shown ind. (d) Replicative senescence is not associated with enhanced autophagy in general. LC3-II expression levels were normalized with β-actin (data inc) and are shown in the bar graphs as relative values to replicatively senescent cells without bafilomycin A1 (S/−; defined as 1). The LC3-II levels in replicatively senescent cells were higher than those in early-passage cells whether in the presence or absence of bafilomycin A1, which may suggest increased synthesis of autophagosomes at replicative senescence7,37. However, the differences in LC3-II levels between the presence and absence of bafilomycin A1 were similar in early-passage and replicatively senescent cells: in MRC-5, 1.9 for Y (2.1−0.2) and 2.0 for S (3.0−1); in WI-38, 1.6 for Y (2.2−0.6) and 1.6 for S (2.6−1). These data indicate that early-passage and replicatively senescent cells have similar rates of autophagic flux, that is, the number of autophagosomes that are delivered to lysosomes for degradation7,37. Figure 1: Pharmacological inhibition of autophagy restores Δ133p53α expression. ( a ) Δ133p53α expression is induced by cycloheximide (CHX). MRC-5 fibroblasts (at population doubling levels (PDLs) 51) were treated with CHX (25 μg ml −1 ) for indicated time periods and examined in immunoblot for Δ133p53α and full-length p53. β-actin was a loading control for normalization. The relative expression levels of Δ133p53α and full-length p53 are shown below the images. ( b ) Δ133p53α expression is induced by phosphoinositide 3-kinase inhibitors. MRC-5 fibroblasts (PDLs 51) were treated for 4 h with LY303511 (10 μM), LY294002 (10 μM), Wortmannin (50 nM) or dimethylsulphoxide alone (as control) and examined in immunoblot for Δ133p53α and β-actin expression. ( c ) Diminished Δ133p53α at replicative senescence is restored by treatment with bafilomycin A1. The immunoblot analyses were performed in early-passage (Y) and replicatively senescent (S) human fibroblast strains MRC-5 and WI-38. The examined PDLs were 30 (Y) and 60 (S) for MRC-5; and 30 (Y) and 54 (S) for WI-38. Bafilomycin A 1 treatment was at 100 nM for 4 h. The relative expression levels of Δ133p53α, full-length p53 and p62/SQSTM1 (normalized with β-actin) are shown. Anti-LC3B antibody detected LC3-I and LC3-II, which was used in quantitative analysis shown in d . ( d ) Replicative senescence is not associated with enhanced autophagy in general. LC3-II expression levels were normalized with β-actin (data in c ) and are shown in the bar graphs as relative values to replicatively senescent cells without bafilomycin A1 (S/−; defined as 1). The LC3-II levels in replicatively senescent cells were higher than those in early-passage cells whether in the presence or absence of bafilomycin A1, which may suggest increased synthesis of autophagosomes at replicative senescence [7] , [37] . However, the differences in LC3-II levels between the presence and absence of bafilomycin A1 were similar in early-passage and replicatively senescent cells: in MRC-5, 1.9 for Y (2.1−0.2) and 2.0 for S (3.0−1); in WI-38, 1.6 for Y (2.2−0.6) and 1.6 for S (2.6−1). These data indicate that early-passage and replicatively senescent cells have similar rates of autophagic flux, that is, the number of autophagosomes that are delivered to lysosomes for degradation [7] , [37] . Full size image For a specific pharmacological inhibition of autophagy, two human fibroblast strains (MRC-5 and WI-38) at early-passage, proliferating phase (Y in Fig. 1c ) and at replicative senescence (S in Fig. 1c ) were treated with bafilomycin A1, which inhibits autophagic flux through specific inhibition of the vacuolar type H(+)-ATPase in lysosomes [7] . As reported [30] , the expression levels of Δ133p53α were diminished in replicatively senescent MRC-5 and WI-38 fibroblasts ( Fig. 1c ; compare Y and S without bafilomycin A1). While the expression of Δ133p53α in early-passage fibroblasts was not significantly changed by bafilomycin A1 treatment ( Fig. 1c ; compare − and + in Y), the same treatment resulted in a striking restoration of Δ133p53α protein levels in replicatively senescent cells ( Fig. 1c ; compare − and + in S). As a control, full-length p53, which is subject to proteasomal degradation [30] , did not significantly change in expression following the bafilomycin A1 treatment in early passage or replicatively senescent fibroblasts ( Fig. 1c ). Although p62/SQSTM1, a known autophagy substrate, was slightly downregulated at replicative senescence, it was stabilized by bafilomycin A1 in both early passage and replicatively senescent cells ( Fig. 1c ), indicating that autophagy functions to degrade this substrate in both of these cells. The quantitation of LC3-II protein amounts in the presence and absence of bafilomycin A1 showed that early passage and replicatively senescent cells had similar rates of autophagic flux (that is, the number of autophagosomes that are delivered to lysosomes for degradation [7] , [37] ) ( Fig. 1d ), suggesting that the autophagic degradation of Δ133p53α during replicative senescence is not due to increased levels of autophagy in general, but due to a regulatory process more specific to Δ133p53α. Knockdown of autophagy-mediating proteins restores Δ133p53α Endogenous expression of pro-autophagic proteins, such as ATG5 ( Fig. 2a ; detected as ATG5–ATG12 conjugate), ATG7 ( Fig. 2b ) and Beclin-1 ( Fig. 2c ), was knocked down via short interfering RNA (siRNA) in MRC-5 fibroblasts approaching replicative senescence. Three independent siRNAs for each protein achieved efficient knockdown and inhibited autophagic activity, as indicated by accumulated LC3-I (ref. 7 ; Fig. 2a–c ). Each siRNA against these three proteins resulted in ~4- to 10-fold higher levels of Δ133p53α protein than control siRNA ( Fig. 2a–d ), while p62/SQSTM1 was similarly increased ( Fig. 2d ) and full-length p53 was not significantly affected ( Fig. 2a–c ), again indicating that autophagic degradation restricts the amounts of Δ133p53α protein but not full-length p53 protein. These siRNAs were less effective in the presence of bafilomycin A1 ( Fig. 2d ), further supporting that their effects were through inhibition of autophagy. Nutrient starvation, which activates autophagy [1] , [7] , also resulted in a time-dependent decrease in Δ133p53α protein exogenously expressed in p53-null fibroblasts ( Supplementary Fig. 1a ), which was abrogated by either bafilomycin A1 treatment or siRNA knockdown of pro-autophagic proteins ( Supplementary Fig. 1b ), suggesting an autophagic regulation of Δ133p53α independent of full-length p53. Taken together, with the above findings from pharmacological inhibition of autophagy, we conclude that the degradation of Δ133p53α via autophagy is responsible for its downregulation during replicative senescence in human fibroblasts. 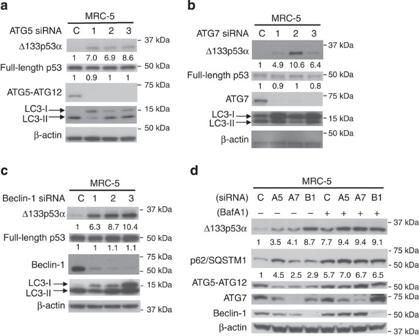Figure 2: siRNA-mediated knockdown of autophagy restores Δ133p53α expression. (a–c) Knockdown of pro-autophagic proteins restores Δ133p53α expression. MRC-5 fibroblasts at late-passage (PDLs 51) were transfected with three independent siRNA oligonucleotides (lanes 1–3) against ATG5 (a), ATG7 (b) and Beclin-1 (c), along with their control siRNA (lane C), for 4 days. Knockdown of ATG5 was confirmed by the loss of ATG5–ATG12 conjugate (detected by anti-ATG5 antibody). Knockdown of the other two proteins was confirmed using the corresponding antibodies. Δ133p53α, full-length p53 and LC3B (LC3-I and LC3-II) were examined in all samples. The relative expression levels of Δ133p53α and full-length p53 (normalized with β-actin) are shown below the images. (d) Knockdown of pro-autophagic proteins and treatment with bafilomycin A1 show similar effects on Δ133p53α and p62/SQSTM1. MRC-5 fibroblasts at late-passage (PDLs 51) were transfected with control siRNA (c), ATG5 siRNA (A5, no. 1 ina), ATG7 siRNA (A7, no. 1 inb) and Beclin-1 siRNA (B1, no. 2 inc) as ina–c, untreated (−) or treated with bafilomycin A1 (+, 100 nM for 4 h), and examined in immunoblots for indicated proteins. The relative expression levels of Δ133p53α and p62/SQSTM1 (normalized with β-actin) are shown below the images. Figure 2: siRNA-mediated knockdown of autophagy restores Δ133p53α expression. ( a – c ) Knockdown of pro-autophagic proteins restores Δ133p53α expression. MRC-5 fibroblasts at late-passage (PDLs 51) were transfected with three independent siRNA oligonucleotides (lanes 1–3) against ATG5 ( a ), ATG7 ( b ) and Beclin-1 ( c ), along with their control siRNA (lane C), for 4 days. Knockdown of ATG5 was confirmed by the loss of ATG5–ATG12 conjugate (detected by anti-ATG5 antibody). Knockdown of the other two proteins was confirmed using the corresponding antibodies. Δ133p53α, full-length p53 and LC3B (LC3-I and LC3-II) were examined in all samples. The relative expression levels of Δ133p53α and full-length p53 (normalized with β-actin) are shown below the images. ( d ) Knockdown of pro-autophagic proteins and treatment with bafilomycin A1 show similar effects on Δ133p53α and p62/SQSTM1. MRC-5 fibroblasts at late-passage (PDLs 51) were transfected with control siRNA ( c ), ATG5 siRNA (A5, no. 1 in a ), ATG7 siRNA (A7, no. 1 in b ) and Beclin-1 siRNA (B1, no. 2 in c ) as in a – c , untreated (−) or treated with bafilomycin A1 (+, 100 nM for 4 h), and examined in immunoblots for indicated proteins. The relative expression levels of Δ133p53α and p62/SQSTM1 (normalized with β-actin) are shown below the images. Full size image E3 ubiquitin ligase STUB1 interacts with Δ133p53α To identify a specific regulator of the autophagic degradation of Δ133p53α, we performed the mass spectrometry analysis of proteins that were co-immunoprecipitated with FLAG-tagged Δ133p53α expressed in MRC-5 fibroblasts, which were either under nutrient starvation with bafilomycin A1 treatment or under normal nutrient-rich conditions (all interacting proteins identified are listed in Supplementary Table 1 ). Of note, peptides from Hsp70 chaperone families (that is, HSPA1A, HSPA1B, HSPA2, HSPA6, HSPA8 and HSPA9) [38] ; the chaperone-associated E3 ubiquitin ligase STUB1 (STIP1 homology and U-Box containing protein 1, also known as CHIP, carboxy terminus of Hsp70-interacting protein) [39] ( Supplementary Fig. 2a ); and Bcl-2-associated athanogene family of chaperone regulators BAG2 (ref. 40 ; Supplementary Fig. 3a ) and BAG5 (ref. 41 ) were identified, suggesting that Δ133p53α is held in the Hsp70 chaperone complex. No peptide sequences from MDM2 were found, consistent with the lack of the major MDM2-interacting region in Δ133p53α (ref. 31 ). Co-immunoprecipitation experiments confirmed the interaction between FLAG-tagged Δ133p53α and STUB1 ( Supplementary Fig. 2b,c ), and suggested that this interaction could occur in the absence of full-length p53 ( Supplementary Fig. 2b ). As STUB1 is a known interactor of Hsp70 chaperones [42] and the C-terminal region of p53 is known to interact with Hsp70 (ref. 43 ), it is possible that the Δ133p53α–STUB1 interaction is indirect through their individual binding to Hsp70 ( Supplementary Fig. 2d ). MDM2 and other E3 ubiquitin ligases interacting with full-length p53 (COP1 and ARFBP1) [44] did not detectably interact with FLAG-Δ133p53α ( Supplementary Fig. 2b,e ). BAG2 ( Supplementary Fig. 3b ), but not BAG5, was also confirmed to interact with FLAG-Δ133p53α. STUB1 is an endogenous regulator of Δ133p53α and senescence The endogenous expression of STUB1 was downregulated in replicatively senescent MRC-5 and WI-38 fibroblasts both at the protein level ( Fig. 3a ) and at the mRNA level ( Fig. 3b ), while early passage and senescent fibroblasts expressed similar levels of BAG2 ( Supplementary Fig. 3c ). The concurrent change in expression of STUB1 and Δ133p53α and their physical interaction prompted us to examine whether STUB1 is a regulator of Δ133p53α expression. The siRNA knockdown of endogenous STUB1 in early-passage MRC-5 fibroblasts resulted in a significant reduction in Δ133p53α with a slight increase in full-length p53 and p62/SQSTM1 ( Fig. 3c ). In contrast, MDM2 knockdown neither downregulated Δ133p53α by itself nor affected the STUB1 knockdown-induced reduction in Δ133p53α ( Supplementary Fig. 4 ), consistent with lack of interaction between MDM2 and Δ133p53α. The cells with STUB1 knockdown showed inhibited proliferation ( Fig. 3d ) with senescence-associated (SA) β-galactosidase (Gal) activity ( Fig. 3e and Supplementary Fig. 5a ), as well as the upregulation of p21 WAF1 as a downstream effector of p53-mediated senescence [27] ( Fig. 3f ) and interleukin (IL)-8 as a SA secretory phenotype [45] ( Fig. 3g ). Thus, inhibition of endogenous STUB1 in early-passage cells reproduced the characteristics of replicatively senescent cells, including diminished expression of Δ133p53α and senescent cellular phenotypes. The lentiviral reconstitution of Δ133p53α expression in the STUB1-knocked down cells, but not transduction with the control vector, restored cell numbers ( Supplementary Fig. 5b ) and abrogated SA-β-Gal activity ( Fig. 3h ), further supporting that the effect of STUB1 on cell proliferation and senescence was through the regulation of Δ133p53α. The STUB1 knockdown did not affect cell proliferation or induce senescence in p53-null MDAH041 −/− fibroblasts ( Supplementary Fig. 6 ). These results indicate that the endogenous level of STUB1 expression is critical to maintain Δ133p53α expression in proliferating cells and that its downregulation leads to diminished expression of Δ133p53α and thereby induction of p53-mediated senescence. The siRNA knockdown or overexpression of BAG2 did not affect Δ133p53α levels ( Supplementary Fig. 3d ), while overexpression of STUB1 in late-passage MRC-5 fibroblasts upregulated Δ133p53α expression ( Supplementary Fig. 2f ). 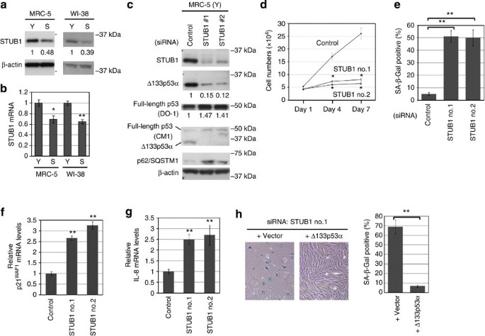Figure 3: Endogenous STUB1 regulates Δ133p53α expression and senescence. (a) Endogenous STUB1 protein is downregulated at replicative senescence. Immunoblot was performed using early-passage (Y) and replicatively senescent (S) fibroblasts (the same set of cells without treatment as inFig. 1c). (b) STUB1 mRNA is downregulated at replicative senescence. The same set of cells as inawere examined by qRT–PCR. Data were from triplicate experiments (mean±s.d.). *P<0.01; **P<0.001 (Student’st-test). (c) Knockdown of STUB1 represses Δ133p53α. MRC-5 fibroblasts (30 PDLs) were transfected with two siRNAs against STUB1 (no. 1 and no. 2) and control siRNA. At 4 days after transfection, immunoblots were performed using anti-STUB1, anti-Δ133p53α, DO-1 (detecting full-length p53), CM1 (detecting both Δ133p53α and full-length p53), anti-p62/SQSTM1 and anti-β-actin antibodies. (d) STUB1 knockdown inhibits cell proliferation. MRC-5 fibroblasts (30 PDLs) were seeded on six-well plates on day 0 (4 × 104cells per well in 6-well plate; nine wells for each siRNA). Cells were counted on days 1, 4 and 7 (three wells each; mean±s.d.), while siRNA transfection was performed on days 1 and 4. *P<0.01 (Student’st-test). (e) STUB1 knockdown induces cellular senescence. The siRNA transfection was performed as incand repeated 4 days later, followed by incubation for 3 days and SA-β-Gal staining. Percentages of SA-β-Gal-positive cells were from triplicate experiments (mean±s.d.). **P<0.001 (Student’st-test). (f,g) STUB1 knockdown upregulates p21WAF1and IL-8. The same set of cells as inewere examined in qRT–PCR for p21WAF1mRNA (f) and IL-8 mRNA (g). Data were from triplicate experiments (mean±s.d.). **P<0.001 (Student’st-test). (h) Δ133p53α rescues STUB1 knockdown-induced senescence. MRC-5 fibroblasts were transfected with STUB1 siRNA (no. 1) as ine. At the next day after the second transfection (on day 5), the cells were transduced with a lentiviral vector driving Δ133p53α or its vector control. At 5 days after the lentiviral transduction, the cells were stained for SA-β-Gal activity. Representative pictures (left) and quantitative data (right) are shown. Percentages of SA-β-Gal-positive cells were from triplicate experiments (mean±s.d.). **P<0.001 (Student’st-test). Figure 3: Endogenous STUB1 regulates Δ133p53α expression and senescence. ( a ) Endogenous STUB1 protein is downregulated at replicative senescence. Immunoblot was performed using early-passage (Y) and replicatively senescent (S) fibroblasts (the same set of cells without treatment as in Fig. 1c ). ( b ) STUB1 mRNA is downregulated at replicative senescence. The same set of cells as in a were examined by qRT–PCR. Data were from triplicate experiments (mean±s.d.). * P <0.01; ** P <0.001 (Student’s t- test). ( c ) Knockdown of STUB1 represses Δ133p53α. MRC-5 fibroblasts (30 PDLs) were transfected with two siRNAs against STUB1 (no. 1 and no. 2) and control siRNA. At 4 days after transfection, immunoblots were performed using anti-STUB1, anti-Δ133p53α, DO-1 (detecting full-length p53), CM1 (detecting both Δ133p53α and full-length p53), anti-p62/SQSTM1 and anti-β-actin antibodies. ( d ) STUB1 knockdown inhibits cell proliferation. MRC-5 fibroblasts (30 PDLs) were seeded on six-well plates on day 0 (4 × 10 4 cells per well in 6-well plate; nine wells for each siRNA). Cells were counted on days 1, 4 and 7 (three wells each; mean±s.d. ), while siRNA transfection was performed on days 1 and 4. * P <0.01 (Student’s t- test). ( e ) STUB1 knockdown induces cellular senescence. The siRNA transfection was performed as in c and repeated 4 days later, followed by incubation for 3 days and SA-β-Gal staining. Percentages of SA-β-Gal-positive cells were from triplicate experiments (mean±s.d.). ** P <0.001 (Student’s t- test). ( f , g ) STUB1 knockdown upregulates p21 WAF1 and IL-8. The same set of cells as in e were examined in qRT–PCR for p21 WAF1 mRNA ( f ) and IL-8 mRNA ( g ). Data were from triplicate experiments (mean±s.d.). ** P <0.001 (Student’s t- test). ( h ) Δ133p53α rescues STUB1 knockdown-induced senescence. MRC-5 fibroblasts were transfected with STUB1 siRNA (no. 1) as in e . At the next day after the second transfection (on day 5), the cells were transduced with a lentiviral vector driving Δ133p53α or its vector control. At 5 days after the lentiviral transduction, the cells were stained for SA-β-Gal activity. Representative pictures (left) and quantitative data (right) are shown. Percentages of SA-β-Gal-positive cells were from triplicate experiments (mean±s.d.). ** P <0.001 (Student’s t- test). Full size image STUB1 protects Δ133p53α from autophagic degradation To examine whether the diminished level of Δ133p53α in STUB1-knocked down cells was due to its autophagic degradation, the siRNA knockdown of STUB1 was performed in combination with treatment with bafilomycin A1 or MG-132. While the inhibition of proteasomal degradation by MG-132 stabilized full-length p53 ( Fig. 4a ), it did not restore the expression level of Δ133p53α in the STUB1-knocked down cells ( Fig. 4a and Supplementary Fig. 7 ), as previously observed in replicatively senescent cells [30] . In contrast, the inhibition of autophagy by bafilomycin A1 remarkably restored Δ133p53α expression with no or little effect on full-length p53 ( Fig. 4a and Supplementary Fig. 7 ), reproducing the findings in replicatively senescent cells ( Fig. 1c ). The inhibition of autophagy by siRNA knockdown of the pro-autophagic proteins also reverted the STUB1 knockdown-induced repression of Δ133p53α ( Fig. 4b ). We next performed co-immunoprecipitation assays to examine whether recruitment of Δ133p53α to autophagosomes involves the senescence-associated degradation of Δ133p53α ( Fig. 4c ). Upon replicative senescence or senescence induced by STUB1 knockdown, the amounts of endogenous Δ133p53α protein interacting with STUB1 were decreased in accordance with decreased STUB1 amounts ( Fig. 4c , IP with anti-STUB1). While Hsp70 levels were maintained, the amounts of Hsp70-interacting Δ133p53α were also decreased with replicative senescence and STUB1 knockdown-induced senescence ( Fig. 4c , IP with anti-Hsp70). In contrast, increased amounts of endogenous Δ133p53α became interacted with an autophagosome component LC3B upon replicative senescence and STUB1 knockdown-induced senescence ( Fig. 4c , IP with anti-LC3B). As expected, treatment with bafilomycin A1 stabilized the LC3B-interacting Δ133p53α protein in these senescent cells ( Fig. 4d ), suggesting that the senescence-associated recruitment of Δ133p53α to autophagosomes leads to its degradation. These results suggest that STUB1 functions to protect Δ133p53α from autophagosome recruitment and autophagic degradation ( Fig. 4e ). 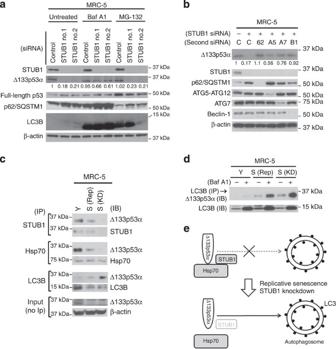Figure 4: STUB1 protects Δ133p53α from autophagic degradation. (a) STUB1 knockdown-induced repression of Δ133p53α is abrogated by bafilomycin A1 treatment. The siRNA transfection in MRC-5 fibroblasts was performed as inFig. 3e. At 7 days after the initial transfection, the cells were untreated, treated with bafilomycin A1 (100 nM for 4 h) or treated with MG-132 (15 μM for 4 h), and examined in immunoblots as indicated. The results of Δ133p53α, full-length p53 and p62/SQSTM1 in untreated cells replicate those shown inFig. 3c. The inhibition of autophagy by bafilomycin A1 was confirmed by increased levels of p62/SQSTM1 and LC3B. The inhibition of proteasomal degradation by MG-132 was confirmed by increased full-length p53. (b) STUB1 knockdown-induced repression of Δ133p53α is abrogated by knockdown of pro-autophagic proteins. MRC-5 fibroblasts (PDLs 30) were transfected for 4 days with control siRNA (−) or STUB1 siRNA (no. 1, +), in combination with control siRNA (c), p62/SQSTM1 siRNA (62), ATG5 siRNA (A5, no. 1 inFig. 2a), ATG7 siRNA (A7, no. 1 inFig. 2b) or Beclin-1 siRNA (B1, no. 2 inFig. 2c), and examined in immunoblots for indicated proteins. (c) Δ133p53α is recruited to autophagosomes upon STUB1 downregulation. MRC-5 fibroblasts at early passage (PDLs 30; Y), those at or close to replicative senescence (PDLs 58; S (Rep)) and those induced to senesce by STUB1 knockdown (S (KD)) were used in immunoprecipitation (IP) with anti-STUB1, anti-Hsp70 and anti-LC3B antibodies, followed by immunoblots (IB) as indicated. Whole-protein lysates without IP (input) were also examined for Δ133p53α and β-actin levels. (d) Bafilomycin A1 stabilizes LC3B-interacting Δ133p53α in senescent cells. The same set of cells as incwere treated with bafilomycin A1 (+, 100 nM for 4 h) or untreated (−). These cells were used in IP with anti-LC3B antibody, followed by IB with anti-Δ133p53 antibody. Whole-protein lysates without IP were also examined in IB with anti-LC3B antibody. While untreated samples replicate the result shown inc, the differences between early passage and senescent cells become more evident with bafilomycin A1 treatment. (e) Schematic model of the regulation of Δ133p53α degradation by STUB1. Figure 4: STUB1 protects Δ133p53α from autophagic degradation. ( a ) STUB1 knockdown-induced repression of Δ133p53α is abrogated by bafilomycin A1 treatment. The siRNA transfection in MRC-5 fibroblasts was performed as in Fig. 3e . At 7 days after the initial transfection, the cells were untreated, treated with bafilomycin A1 (100 nM for 4 h) or treated with MG-132 (15 μM for 4 h), and examined in immunoblots as indicated. The results of Δ133p53α, full-length p53 and p62/SQSTM1 in untreated cells replicate those shown in Fig. 3c . The inhibition of autophagy by bafilomycin A1 was confirmed by increased levels of p62/SQSTM1 and LC3B. The inhibition of proteasomal degradation by MG-132 was confirmed by increased full-length p53. ( b ) STUB1 knockdown-induced repression of Δ133p53α is abrogated by knockdown of pro-autophagic proteins. MRC-5 fibroblasts (PDLs 30) were transfected for 4 days with control siRNA (−) or STUB1 siRNA (no. 1, +), in combination with control siRNA ( c ), p62/SQSTM1 siRNA (62), ATG5 siRNA (A5, no. 1 in Fig. 2a ), ATG7 siRNA (A7, no. 1 in Fig. 2b ) or Beclin-1 siRNA (B1, no. 2 in Fig. 2c ), and examined in immunoblots for indicated proteins. ( c ) Δ133p53α is recruited to autophagosomes upon STUB1 downregulation. MRC-5 fibroblasts at early passage (PDLs 30; Y), those at or close to replicative senescence (PDLs 58; S (Rep)) and those induced to senesce by STUB1 knockdown (S (KD)) were used in immunoprecipitation (IP) with anti-STUB1, anti-Hsp70 and anti-LC3B antibodies, followed by immunoblots (IB) as indicated. Whole-protein lysates without IP (input) were also examined for Δ133p53α and β-actin levels. ( d ) Bafilomycin A1 stabilizes LC3B-interacting Δ133p53α in senescent cells. The same set of cells as in c were treated with bafilomycin A1 (+, 100 nM for 4 h) or untreated (−). These cells were used in IP with anti-LC3B antibody, followed by IB with anti-Δ133p53 antibody. Whole-protein lysates without IP were also examined in IB with anti-LC3B antibody. While untreated samples replicate the result shown in c , the differences between early passage and senescent cells become more evident with bafilomycin A1 treatment. ( e ) Schematic model of the regulation of Δ133p53α degradation by STUB1. Full size image Δ133p53α is ubiquitinated for degradation Selective autophagy, as well as proteasome-mediated degradation, involves ubiquitination of substrate proteins [3] , [4] . To examine whether Δ133p53α protein is ubiquitinated, FLAG-tagged Δ133p53α was expressed in MRC-5 fibroblasts under starvation conditions with bafilomycin A1, immunoprecipitated with anti-ubiquitin antibody and then analysed by immunoblot with anti-FLAG antibody ( Fig. 5a ). The cells expressing FLAG-Δ133p53α ( Fig. 5a , lane 2), but not those with vector control ( Fig. 5a , lane 1), showed a smear signal extending over 250 kDa, suggestive of polyubiquitination of Δ133p53α protein. A similar immunoprecipitation (anti-ubiquitin antibody)-immunoblot (anti-Δ133p53 antibody) experiment using untransduced MRC-5 fibroblasts also detected a smear signal derived from endogenous Δ133p53α protein ( Supplementary Fig. 8 ). When FLAG-Δ133p53α expressed in MRC-5 fibroblasts was immunoprecipitated with anti-FLAG antibody and analysed using mass spectrometry, the lysine residues at amino acid positions 248 and 249 were identified to be ubiquitinated ( Fig. 5b ), which correspond to positions 381 and 382 in full-length p53, two of its major ubiquitination sites [44] . The mutation of these two lysine residues ( Fig. 5c ) abrogated the smear signal ( Fig. 5a , lane 4), confirming that it indeed represented polyubiquitinated Δ133p53α and that these lysine residues are the major ubiquitination sites of Δ133p53α. The siRNA knockdown of STUB1 reduced the amount of polyubiquitinated Δ133p53α ( Fig. 5a , lane 3), indicating that this E3 ubiquitin ligase functions to ubiquitinate Δ133p53α. However, a significant amount of residual polyubiquitinated Δ133p53α even with almost complete knockdown of STUB1 suggests that another unidentified E3 ligase may also contribute to Δ133p53α ubiquitination. Importantly, the mutant version of FLAG-Δ133p53α became resistant to starvation- and STUB1 knockdown-induced degradation ( Fig. 5d ), indicating that the ubiquitination of Δ133p53α is essential to its autophagic degradation. 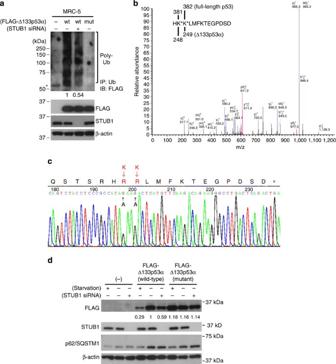Figure 5: Δ133p53α is ubiquitinated for degradation. (a) Δ133p53α protein is polyubiquitinated. FLAG-tagged versions of wild-type Δ133p53α (wt) and mutant Δ133p53α (mut; fromcbelow), along with vector control (−), were retrovirally transduced into MRC-5 fibroblasts. The wild-type Δ133p53α-expressing cells had a pair of STUB1 siRNA-transfected (+, siRNA no. 1 for 4 days) and untransfected (−) counterparts. These cells were maintained for 8 h under amino acid- and serum-starved conditions with bafilomycin A1 (100 nM). Protein lysates were used either in IP with anti-ubiquitin (Ub) antibody, followed by IB with anti-FLAG antibody (top), or directly in IB for FLAG-Δ133p53α, STUB1 and β-actin (lower three panels). Smear signals indicate polyubiquitinated FLAG-Δ133p53α protein (Poly-Ub). Asterisk indicates a nonspecific band in negative control. These experimental conditions resulted in similar amounts of FLAG-Δ133p53α in the presence and absence of STUB1 knockdown, allowing quantitative analysis of ubiquitination. The relative densitometric values of wild-type FLAG-Δ133p53α polyubiquitination in the presence and absence of STUB1 knockdown (normalized with total FLAG-Δ133p53α) are shown. (b) Δ133p53α is ubiquitinated at the C-terminal lysine residues. MRC-5 fibroblasts expressing wild-type FLAG-Δ133p53α in the absence of STUB1 knockdown were used in IP with anti-FLAG antibody, and the resulting immunoprecipitates were analysed using mass spectrometry. Representative MS/MS spectrum of an [M+3H]3+ peptide from FLAG-Δ133p53α shows sites of ubiquitin modification. The peptide sequence for the spectrum is shown, with the sites of modification marked as asterisks: amino-acid positions 248 and 249, which correspond to positions 381 and 382 in full-length p53. The same peptide was also observed in the unmodified state. (c) Lysine (K)-to-arginine (R) substitutions at amino-acid residues 248 and 249. (d) Mutation of the ubiquitination sites renders Δ133p53α resistant to degradation. The same three cells as inawere cultured under amino-acid- and serum-starved conditions for 8 h (without bafilomycin A1), transfected with STUB1 siRNA (no. 1 for 4 days) or untreated, and examined in IBs for FLAG-Δ133p53α, STUB1, p62/SQSTM1 and β-actin. The effect of starvation was confirmed by decreased p62/SQSTM1 in each cell. The upregulation of p62/SQSTM1 by wild-type and mutant FLAG-Δ133p53α is likely associated with enhanced cell proliferation by Δ133p53α overexpression30. Figure 5: Δ133p53α is ubiquitinated for degradation. ( a ) Δ133p53α protein is polyubiquitinated. FLAG-tagged versions of wild-type Δ133p53α (wt) and mutant Δ133p53α (mut; from c below), along with vector control (−), were retrovirally transduced into MRC-5 fibroblasts. The wild-type Δ133p53α-expressing cells had a pair of STUB1 siRNA-transfected (+, siRNA no. 1 for 4 days) and untransfected (−) counterparts. These cells were maintained for 8 h under amino acid- and serum-starved conditions with bafilomycin A1 (100 nM). Protein lysates were used either in IP with anti-ubiquitin (Ub) antibody, followed by IB with anti-FLAG antibody (top), or directly in IB for FLAG-Δ133p53α, STUB1 and β-actin (lower three panels). Smear signals indicate polyubiquitinated FLAG-Δ133p53α protein (Poly-Ub). Asterisk indicates a nonspecific band in negative control. These experimental conditions resulted in similar amounts of FLAG-Δ133p53α in the presence and absence of STUB1 knockdown, allowing quantitative analysis of ubiquitination. The relative densitometric values of wild-type FLAG-Δ133p53α polyubiquitination in the presence and absence of STUB1 knockdown (normalized with total FLAG-Δ133p53α) are shown. ( b ) Δ133p53α is ubiquitinated at the C-terminal lysine residues. MRC-5 fibroblasts expressing wild-type FLAG-Δ133p53α in the absence of STUB1 knockdown were used in IP with anti-FLAG antibody, and the resulting immunoprecipitates were analysed using mass spectrometry. Representative MS/MS spectrum of an [M+3H]3+ peptide from FLAG-Δ133p53α shows sites of ubiquitin modification. The peptide sequence for the spectrum is shown, with the sites of modification marked as asterisks: amino-acid positions 248 and 249, which correspond to positions 381 and 382 in full-length p53. The same peptide was also observed in the unmodified state. ( c ) Lysine (K)-to-arginine (R) substitutions at amino-acid residues 248 and 249. ( d ) Mutation of the ubiquitination sites renders Δ133p53α resistant to degradation. The same three cells as in a were cultured under amino-acid- and serum-starved conditions for 8 h (without bafilomycin A1), transfected with STUB1 siRNA (no. 1 for 4 days) or untreated, and examined in IBs for FLAG-Δ133p53α, STUB1, p62/SQSTM1 and β-actin. The effect of starvation was confirmed by decreased p62/SQSTM1 in each cell. The upregulation of p62/SQSTM1 by wild-type and mutant FLAG-Δ133p53α is likely associated with enhanced cell proliferation by Δ133p53α overexpression [30] . Full size image Δ133p53α is colocalized with p62/SQSTM1 and LC3B The p62/SQSTM1-mediated recruitment to autophagosomes is another characteristic of selective autophagy substrates. To examine whether Δ133p53α is colocalized with p62/SQSTM1, epitope-tagged versions of Δ133p53α (V5 tag or FLAG tag) were expressed in MRC-5 fibroblasts because the current anti-Δ133p53 antibody does not work in immunofluorescence cell staining. While Δ133p53α was shown to be localized in the nucleus, as previously reported [28] , [30] , under standard nutrient-rich culture condition, autophagy induction by nutrient starvation induced the formation of discrete cytoplasmic foci and aggregates of Δ133p53α ( Supplementary Fig. 9a ). These cytoplasmic Δ133p53α foci and aggregates were colocalized with p62/SQSTM1 (FLAG tag in Fig. 6a , V5 tag in Supplementary Fig. 9b ). The cytoplasmic colocalization of Δ133p53α with p62/SQSTM1 was also induced by siRNA knockdown of STUB1 ( Supplementary Fig. 9c ). A co-immunoprecipitation experiment using FLAG-Δ133p53α-expressing MRC-5 fibroblasts confirmed the physical interaction of Δ133p53α with p62/SQSTM1 ( Supplementary Fig. 9d ). Furthermore, siRNA knockdown of p62/SQSTM1 resulted in restored expression of endogenous Δ133p53α in late-passage MRC-5 fibroblasts ( Fig. 6b ) and STUB1-knocked down MRC-5 fibroblasts ( Fig. 4b ), suggesting the functional involvement of p62/SQSTM1 in Δ133p53α degradation via selective autophagy. The starvation- and STUB1 knockdown-induced cytoplasmic Δ133p53α foci and aggregates were confirmed to be colocalized with LC3B as well (FLAG tag in Fig. 6c,d , V5 tag in Supplementary Fig. 9e,f ), consistent with the recruitment of endogenous Δ133p53α to autophagosomes at replicative senescence and STUB1 knockdown-induced senescence ( Fig. 4c,d ). 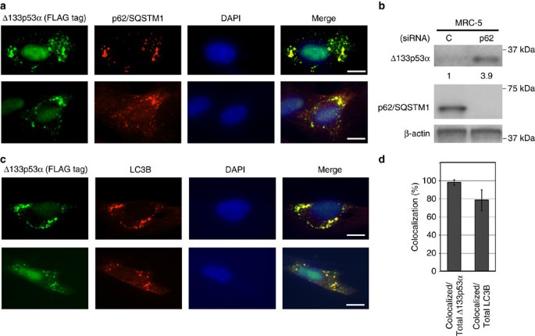Figure 6: Δ133p53α is colocalized with p62/SQSTM1 and LC3B. (a) Δ133p53α is colocalized with p62/SQSTM1 upon autophagy induction. MRC-5 fibroblasts expressing FLAG-Δ133p53α (wild-type) were cultured under amino-acid- and serum-starved conditions for 4 h, and co-immunostained with anti-FLAG antibody (Δ133p53α, green) and anti-p62/SQSTM1 antibody (red). Two representative sets of images, including nuclear staining with 4′,6-diamidino-2-phenylindole (DAPI) and merged images, are shown. Scale bars, 10 μm. (b) Knockdown of p62/SQSTM1 stabilizes endogenous Δ133p53α. MRC-5 fibroblasts at late passage (PDLs 51) were transfected with p62/SQSTM1 siRNA (p62) or control siRNA (C) for 3 days, and examined in immunoblots for Δ133p53α and p62/SQSTM1 expression. The relative expression levels of Δ133p53α (normalized with β-actin) are shown. (c) Δ133p53α is colocalized with LC3B upon autophagy induction. MRC-5 fibroblasts with FLAG-Δ133p53α under starved conditions (as ina) were co-immunostained with anti-FLAG antibody (Δ133p53α, green) and anti-LC3B antibody (red). Two representative sets of images, including DAPI and merged images, are shown. Scale bars, 10 μm. (d) Quantitative analysis of Δ133p53α-LC3B colocalization. The number of colocalized signals out of total number of Δ133p53α signals or out of total number of LC3B signals was counted in 26 cells. Data (percent colocalization) are mean±s.d. Almost all Δ133p53α signals were colocalized with LC3B, while ~80% of LC3B signals were colocalized with Δ133p53α. Figure 6: Δ133p53α is colocalized with p62/SQSTM1 and LC3B. ( a ) Δ133p53α is colocalized with p62/SQSTM1 upon autophagy induction. MRC-5 fibroblasts expressing FLAG-Δ133p53α (wild-type) were cultured under amino-acid- and serum-starved conditions for 4 h, and co-immunostained with anti-FLAG antibody (Δ133p53α, green) and anti-p62/SQSTM1 antibody (red). Two representative sets of images, including nuclear staining with 4′,6-diamidino-2-phenylindole (DAPI) and merged images, are shown. Scale bars, 10 μm. ( b ) Knockdown of p62/SQSTM1 stabilizes endogenous Δ133p53α. MRC-5 fibroblasts at late passage (PDLs 51) were transfected with p62/SQSTM1 siRNA (p62) or control siRNA (C) for 3 days, and examined in immunoblots for Δ133p53α and p62/SQSTM1 expression. The relative expression levels of Δ133p53α (normalized with β-actin) are shown. ( c ) Δ133p53α is colocalized with LC3B upon autophagy induction. MRC-5 fibroblasts with FLAG-Δ133p53α under starved conditions (as in a ) were co-immunostained with anti-FLAG antibody (Δ133p53α, green) and anti-LC3B antibody (red). Two representative sets of images, including DAPI and merged images, are shown. Scale bars, 10 μm. ( d ) Quantitative analysis of Δ133p53α-LC3B colocalization. The number of colocalized signals out of total number of Δ133p53α signals or out of total number of LC3B signals was counted in 26 cells. Data (percent colocalization) are mean±s.d. Almost all Δ133p53α signals were colocalized with LC3B, while ~80% of LC3B signals were colocalized with Δ133p53α. Full size image This study shows that Δ133p53α, an endogenous regulator of replicative cellular senescence [30] , is degraded by autophagy ( Figs 1 and 2 ), providing a novel functional and regulatory link between cellular senescence and autophagy, two cellular phenotypes involved in aging and cancer [11] , [16] , [19] . Our data also indicate that a specific regulatory mechanism involving STUB1 controls the autophagic degradation of Δ133p53α ( Figs 3 and 4 ) and that Δ133p53α has characteristics of a substrate of selective autophagy ( Figs 5 and 6 ). STUB1 was identified to form a complex with Δ133p53α, while there was no evidence for an interaction between MDM2 and Δ133p53α. STUB1 functionally cooperates with MDM2 to induce proteasomal degradation of full-length p53 (ref. 39 ), which is consistent with slightly increased levels of full-length p53 in response to STUB1 knockdown ( Figs 3c and 4a ). However, our data suggest that STUB1 functions in a different manner to regulate the protein turnover of Δ133p53α, which is not subject to proteasomal degradation ( Fig. 4a ) [30] , does not interacts with MDM2 ( Supplementary Fig. 2b,e ) and is not ubiquitinated by MDM2 (ref. 46 ). Given that STUB1 can act as a molecular switch between proteasomal and lysosomal protein degradation pathways [47] , our data suggest that STUB1 regulates not only proteasomal degradation but also autophagic degradation of substrate proteins, and that the latter activity becomes evident for Δ133p53α in the absence of MDM2-mediated proteasomal degradation. Although Δ133p53α interacts with Hsp70 chaperones and the associated factors including STUB1 ( Supplementary Fig. 2 and Supplementary Table 1 ), Δ133p53α degradation is unlikely to be via chaperone-mediated autophagy [48] , [49] , [50] , [51] , which is independent of ubiquitination, p62/SQSTM1 and autophagosomes (contrary to data shown in Figs 4 , 5 , 6 , Supplementary Figs 8 and 9 ) and is not affected by wortmannin or LY294002 (contrary to data shown in Fig. 1b ). Our findings rather support that the degradation of Δ133p53α falls into a category of chaperone-assisted selective autophagy, for which Hsp70 chaperones, STUB1, ubiquitinated substrate, p62/SQSTM1 and autophagosomes are essential [52] . We hypothesize that, while the formation of the STUB1/Hsp70/Δ133p53α complex may be a prerequisite for Δ133p53α degradation, STUB1 in this complex functions to restrict Δ133p53α degradation by preventing Δ133p53α from being recruited to autophagosomes ( Fig. 4e , top). Consistent with this hypothesis, STUB1 downregulation, whether physiologically during replicative senescence or experimentally by siRNA knockdown, resulted in dissociation of Δ133p53α from Hsp70 and its recruitment to autophagosomes ( Fig. 4c–e , bottom). STUB1 takes part in ubiquitinating Δ133p53α ( Fig. 5a ), consistent with the ability of STUB1 to ubiquitinate full-length p53 (ref. 39 ). However, the partial inhibition of Δ133p53α ubiquitination in the absence of STUB1 ( Fig. 5a ) also suggests that, when STUB1 is downregulated, an unidentified E3 ligase(s) may ubiquitinate Δ133p53α to render it committed to degradation via selective autophagy. Two recent studies [53] , [54] showed that mutant p53 proteins are also degraded by autophagy. Glucose restriction in cancer cells induced MDM2-mediated ubiquitination and autophagic degradation of mutant p53 (ref. 54 ), which is in contrast to no involvement of MDM2 in Δ133p53α degradation. The degradation of mutant p53 via chaperone-mediated autophagy was induced by suppression of macroautophagy (such as by siRNA knockdown of Beclin-1 and ATG proteins) [53] , whereas the same siRNA knockdown inhibited Δ133p53α degradation ( Fig. 2 ). It is interesting to further investigate similarities and differences in protein degradation mechanisms between Δ133p53α and mutant p53, which may be related to their functional similarities and differences. The downregulation of endogenous STUB1 at replicative senescence ( Fig. 3a,b ) and the senescent phenotypes induced by knockdown of endogenous STUB1 ( Fig. 3c–h ) highlight the physiological role of STUB1 in the regulation of cellular senescence. These data are consistent with the previous in vivo studies showing an age-dependent downregulation of STUB1 expression in mouse brain [55] and accelerated aging phenotypes in STUB1-deficient mice [56] . Furthermore, a public microarray data set (GSE19205) [57] available at GEO ( http://www.ncbi.nlm.nih.gov/geo/ ) shows that STUB1 is downregulated in patients of Werner syndrome, a progeroid syndrome with premature aging phenotypes, suggesting its in vivo role in aging in humans as well. Another GEO data set (GDS2534) shows that STUB1 mRNA expression is largely dependent on p63, a member of the p53 family of proteins, which raises a hypothesis that altered transcriptional activity of p63 may be involved in STUB1 downregulation at the mRNA level during replicative senescence. A possible feedback regulation involving p63, STUB1, Δ133p53α and full-length p53 is an interesting subject of future study. While the generation of protein isoforms through initiation of transcription from alternative promoters, alternative mRNA splicing and alternative initiation of translation has been extensively investigated for many human genes [29] , [58] , [59] , little is known about a possible difference in protein degradation mechanisms among protein isoforms. This study is the first demonstration of an isoform-specific autophagic degradation that coordinates a biological process. The differential degradation kinetics between full-length p53 and Δ133p53α would enable efficient induction of p53-mediated replicative senescence. With the autophagic degradation of Δ133p53α and release from its inhibitory effect, maintained levels of full-length p53 with its activation as indicated by serine 15 phosphorylation [30] , [60] could fully induce the p53 target genes responsible for cellular senescence (for example, p21 WAF1 ) [27] and SA secretory phenotype (for example, IL-8) [45] . Indeed, forced expression of Δ133p53α in fibroblasts approaching replicative senescence resulted in a significant delay in the onset of senescent phenotypes [30] . Together with our previous report that the downregulation of the splicing factor SRSF3 induces the alternative RNA splicing generating p53β (a p53 isoform cooperating with full-length p53) during replicative senescence [61] , our findings support the hypothesis that multiple p53 isoforms under different regulatory controls constitute a regulatory network to modulate the functions of full-length p53 in p53-mediated biological processes. p62/SQSTM1 is a substrate of selective autophagy whose roles in aging and cancer have been characterized. The accumulation of p62/SQSTM1 due to defective autophagy activates the proinflammatory transcription factor NF-kB and the stress-responsive transcription factor NRF2 to induce inflammation and tissue injury, which accelerate the aging process [11] , [62] . The p62/SQSTM1-induced activation of these transcription factors also promotes tumour initiation through enhanced cell survival, reactive oxygen species production, chronic inflammation and genome instability [2] , [63] . Our findings in this study have identified Δ133p53α as a novel substrate of selective autophagy, which functions in the p53 signalling network to regulate aging and cancer. Δ133p53α and p62/SQSTM1 showed different susceptibilities to autophagic degradation in early passage and replicatively senescent fibroblasts ( Fig. 1c ). In contrast to the upregulation of both Δ133p53α and p62/SQSTM1 by general inhibition of autophagy ( Fig. 2d ), STUB1 knockdown downregulated Δ133p53α but upregulated p62/SQSTM1 through a currently unknown mechanism ( Figs 3c and 4a ). These results indicate that the degradation of these two autophagy substrates is each under specific control. This study thus opens up a new aspect of autophagy regulation of aging and cancer and highlights the importance of further identification of selective autophagy substrates of different functions. Lastly, given that in vivo downregulation of Δ133p53α in senescent CD8 + T lymphocytes also involves autophagy [64] and that autophagy is a cellular phenotype evolutionarily conserved from unicellular organisms to mammals [11] , our findings from in vitro cultured cells have implications in understanding and manipulating aging and carcinogenesis processes in vivo. Cells, cell treatment and SA-β-Gal staining Normal human fibroblasts MRC-5 and WI-38 were from American Type Culture Collection (Manassas, VA, USA). MDAH041 −/− (p53-null immortalized fibroblast cell line) was provided by M. Tainsky (Case Western Reserve University). Bafilomycin A1, MG-132, cycloheximide and wortmannin were from Sigma-Aldrich (St Louis, MO, USA). LY294002 and LY303511 were from Santa Cruz Biotechnology (Santa Cruz, CA, USA). For amino acid and serum starvation, cells were cultured in MEM Eagle medium with Earle’s and without amino acids (US Biological, M3859-01). SA-β-Gal staining used the Senescence β-Galactosidase Staining Kit (Cell Signaling Technology, Danvers, MA, USA). Vectors and transduction pQCXIN-FLAG-Δ133p53α and pQCXIN-FLAG-p53β were generated by Fujita et al. [30] The truncated versions of pQCXIN-FLAG-Δ133p53α, that is, Tr.1(133–346), Tr.2(133–322) and Tr.3(133–254), were made by restriction digestion of the plasmid with StuI, PflMI and XcmI, respectively, in combination with EcoRI, followed by blunt ending and self-circularization. Two amino-acid substitutions were generated in pQCXIN-FLAG-Δ133p53α (lysine to arginine at amino-acid positions 248 and 249, which correspond to 381 and 382 in full-length p53) by site-directed mutagenesis using the QuikChange II XL kit (Stratagene, Carlsbad, CA, USA). V5-tagged Δ133p53α was expressed from pLenti6/V5-D-TOPO (Invitrogen, Carlsbad, CA, USA). Δ133p53α expression was also driven from pLOC (Open Biosystems, Huntsville, AL, USA), a lentiviral expression vector carrying a green fluorescent protein expression unit. The STUB1 and BAG2 lentiviral expression vectors, as well as the control vector, were purchased from Open Biosystems. Retroviral and lentiviral transduction was carried out using the ViraPort retroviral gene expression system (Agilent Technologies, Santa Clara, CA, USA), the ViraPower lentiviral expression system (Invitrogen) or Trans-lentiviral packaging system (Open Biosystems). Transfection of siRNA oligonucleotides siRNA oligonucleotides were transfected at a final concentration of 12 nM using Lipofectamine RNAiMAX (Invitrogen). When two different siRNAs were co-transfected, their final concentration was 6 nM each. The following oligonucleotides were from Invitrogen: Stealth Select siRNAs targeting ATG5 (no. 1; 5′-GGUUUGGACGAAUUCCAACUUGUUU-3′, no. 2; 5′-GAUCACAAGCAACUCUGGAUGGGAU-3′ and no. 3; 5′-GCCAUCAAUCGGAAACUCAUGGAAU-3′); BECN1 (no. 1; 5′-CCACUCUGUGAGGAAUGCACAGAUA-3′, no. 2; 5′-GGAUGAUGAGCUGAAGAGUGUUGAA-3′ and no. 3; 5′-ACAGUGAAUUUAAACGACAGCAGCU-3′); ATG7 (no. 1; 5′-GCCGUCAUUGCUGCAAGCAAGAGAA-3′, no. 2; 5′-UCUUCGAAGUGAAGCUUCCAGAAAU-3′ and no. 3; 5′-CCAAUCCUGUGAGGAAGCCUCUCUA-3′); STUB1 (no. 1; 5′-GGCAAUCGUCUGUUCGUGGGCCGAA-3′ and no. 2; 5′-CCAGCGCUCUUCGAAUCGCGAAGAA-3′); MDM2 (no. 1; 5′-UAGUUGACCUGUCUAUAAGAGAAUU-3′ and no. 2; 5′-UCUGUACCUACUGAUGGUGCUGUAA-3′); p62/SQSTM1 (5′-AGAAGUGGACCCGUCUACAGGUGAA-3′), Stealth RNAi Negative Control (no. 12,935–100); Silencer Select siRNAs targeting BAG2 (no. 1; 5′-GCAAGAAUCCCUAAAGCAU-3′ and no. 2; 5′-GCUGUGCUCUUGAAGAUCA-3′); and Silencer Select Negative Control (no. 4390843). Immunoblot Protein lysates (30–50 μg per sample) were separated on 10 or 4–20% gradient SDS-polyacrylamide gels (Invitrogen) and transferred to Hybond-P PVDF membranes (GE HealthCare Life Sciences, Pittsburgh, PA, USA). Incubations with primary and secondary antibodies and signal detection followed the suppliers’ protocol using ECL western blotting detection system (GE HealthCare Life Sciences) or SuperSignal West Dura chemiluminescent substrate (Thermo Scientific, Westminster, MD, USA). Quantitative image analysis was performed using the ImageJ 1.40g software ( http://rsb.info.nih.gov/ij/ ). The following primary antibodies were used in immunoblot: anti-p53 (1:2,000; DO-1, Santa Cruz Biotechnology); anti-p53 (1:1,000; CM1, Signet Laboratories, Dedham, MA, USA); anti-FLAG (1:5,000; M2, Sigma-Aldrich); anti-FLAG M2-peroxidase (horseradish peroxidase; 1:1,000; A8592, Sigma-Aldrich); anti-polyubiquitin (1:500; P4D1, Santa Cruz Biotechnology); anti-ATG5 (1:5,000; no. 2,630, Cell Signaling Technology); anti-Beclin-1 (1:2,000; no. 3,788, Cell Signaling Technology); anti-ATG7 (1:5,000; PM039, MBL); anti-p62/SQSTM1 (1:5,000; PM045, MBL); anti-LC3B (1:1,000; M152-3, MBL); anti-STUB1 (1:1,000; S1073, Sigma-Aldrich); anti-BAG2 (1:2,000; ab47106, Abcam); anti-COP1 (1:5,000; A300–894, Bethyl Lab); anti-ARFBP1 (1:2,000; ab70161, Abcam); anti-MDM2 (1:500; sc-965, Santa Cruz Biotechnology); anti-Hsp70 (1:1,000; MA3–007, Thermo Scientific) and anti-β-actin (1:10,000; AC-15, Sigma-Aldrich). Anti-Δ133p53 antibody (1:5,000; MAP4, rabbit polyclonal) was used by Fujita et al. [30] and Mondal et al. [64] Note that MAP4 works in immunoblot to detect ~35-kDa band of Δ133p53α with some nonspecific bands [30] , [64] , but does not work in immunoprecipitation or immunofluorescence staining (in which FLAG- or V5-tagged Δ133p53α protein and corresponding antibodies were used). Horseradish peroxidase-conjugated goat anti-mouse and anti-rabbit antibodies (Santa Cruz Biotechnology) were used as secondary antibodies. Immunoprecipitation Protein lysates were prepared in 50 mM Tris-HCl (pH 7.5)/150 mM NaCl/1 mM EDTA/1% NP-40 with protease inhibitors and were used for immunoprecipitation (500 μg per sample) at 4 °C overnight with 10 μg of the following antibodies: anti-FLAG M2 affinity gel (F2426, Sigma-Aldrich); anti-polyubiquitin (P4D1, agarose-conjugated, Santa Cruz Biotechnology); anti-STUB1 (12A11, MBL); anti-Hsp70 (5A5, Thermo Scientific) and anti-LC3B (SAB4200361, Sigma-Aldrich). Twenty microlitres of bed volume of Protein G Plus-agarose (Santa Cruz Biotechnology) were included in incubation with anti-STUB1, anti-Hsp70 and anti-LC3B antibodies. The resulting immunoprecipitates were analysed using immunoblot as above. Real-time quantitative reverse transcription–PCR (qRT–PCR) RNA samples were prepared using TRIzol (Invitrogen) and reverse-transcribed by SuperScript III 1st strand synthesis system (Invitrogen). For real-time qRT–PCR reaction, Taqman universal PCR master mix (Applied Biosystems) was used with the following primers/probe sets purchased from Applied Biosystems: STUB1 (Hs01071598_g1); IL-8 (Hs00174103_m1) and p21 WAF1 (Hs99999142_m1). The endogenous control was GAPDH (Hs03929097_g1). The quantitative data analysis was performed according to the supplier’s protocol (Applied Biosystems, protocol no. 4310255B). Immunofluorescence staining Cells were grown on Lab-Tek II chamber slides (Nalge Nunc International, Rochester, NY, USA), fixed with 2% paraformaldehyde and permeabilized with 0.2% Triton X-100. Immunofluorescence staining was performed using anti-FLAG (1:500; M2, Sigma-Aldrich), anti-V5 (1:200; P/N46-0705, Invitrogen), anti-p62/SQSTM1 (1:500; PM045, MBL) and anti-LC3B (1:400; no. 2,775, Cell Signaling Technology) antibodies. Alexa 488- or Alexa 568-conjugated goat anti-mouse and anti-rabbit antibodies (Invitrogen) were secondary antibodies. The slides were mounted with ProLong Gold antifade reagent with 4′,6-diamidino-2-phenylindole (Invitrogen). Mass spectrometry Immunoprecipitates with anti-FLAG antibody from MRC-5 fibroblasts expressing FLAG-tagged Δ133p53α, either under normal nutrient-rich conditions or under nutrient starvation with bafilomycin A1 treatment, were analysed using mass spectrometry. The immunoprecipitates were separated on a 4–12% Bis-Tris gel and stained with Colloidal Coomassie (Invitrogen). The band corresponding to the FLAG-Δ133p53α and multiple bands at higher molecular weight were cut from the gel and subjected to in-gel reduction with dithiothreitol (DTT) and alkylation with iodoacetamide. The proteins were then digested with endoproteinase ArgC (Protea Biosciences, Morgantown, WV, USA) in 50 mM ammonium bicarbonate, 20 mM calcium acetate, 2.5 mM DTT for 20 h at 25 °C. The resulting peptides were extracted and dried by vacuum evaporation. Mass spectrometry analysis was performed using an LTQ ion trap mass spectrometer (Thermo Scientific) equipped with an ADVANCE CaptiveSpray ion source (Michrom Bioresources, Auburn, CA, USA). Peptides were separated on a 0.2 × 50 mm Magic C18AQ reverse phase column (Michrom Bioresources) using the Paradigm MS4 HPLC (Michrom Bioresources) at a flow rate of 2 μl min −1 followed by online analysis using tandem mass spectrometry. Spectra were searched against the human IPI database (v 3.72) using TurboSEQUEST in BioWorks v. 3.3.1 SP1 (ThermoElectron, San Jose, CA, USA). The search parameters included: precursor mass tolerance: ±1.5 a.m.u. ; fragment mass tolerance: ±0.8 a.m.u. ; a static modification of +57.02 on cysteine; a variable modification of +15.99 for methionine oxidation; a variable modification of +114.04 on lysine for GG modification that remains after cleavage of conjugated ubiquitin [65] . Statistical analyses Student’s t- test was used. How to cite this article: Horikawa, I. et al. Autophagic degradation of the inhibitory p53 isoform Δ133p53α as a regulatory mechanism for p53-mediated senescence. Nat. Commun. 5:4706 doi: 10.1038/ncomms5706 (2014).